Adaptive introgression betweenAnophelessibling species eliminates a major genomic island but not reproductive isolation Adaptive introgression can provide novel genetic variation to fuel rapid evolutionary responses, though it may be counterbalanced by potential for detrimental disruption of the recipient genomic background. We examine the extent and impact of recent introgression of a strongly selected insecticide-resistance mutation ( Vgsc-1014F ) located within one of two exceptionally large genomic islands of divergence separating the Anopheles gambiae species pair. Here we show that transfer of the Vgsc mutation results in homogenization of the entire genomic island region (~1.5% of the genome) between species. Despite this massive disruption, introgression is clearly adaptive with a dramatic rise in frequency of Vgsc-1014F and no discernable impact on subsequent reproductive isolation between species. Our results show (1) how resilience of genomes to massive introgression can permit rapid adaptive response to anthropogenic selection and (2) that even extreme prominence of genomic islands of divergence can be an unreliable indicator of importance in speciation. Anthropogenic habitat changes present a difficult evolutionary challenge for both intentionally and unintentionally targeted organisms, because of the speed at which they occur. Introgressive hybridization between incompletely reproductively isolated species provides a mechanism for the rapid acquisition of novel genetic variation which can accelerate adaptive evolution and is of recognized importance for plants [1] . However, only a few clear cases have been demonstrated in animals, for example, the transfer of rodenticide tolerance between mouse species [2] and of wing colour patterns among Heliconius butterflies [3] , [4] . A major obstacle to adaptive introgression is the rate at which recombination can separate beneficial genetic variants within an introgressed fragment from the wider donor background. The disruptive effect of this perturbation of epistasis within the recipient species genome is likely to be deleterious [5] . This may be exacerbated if introgressed adaptive variants are located in low recombination regions, because the hitchhiked portions of the donor species’ genome will take longer to eliminate. Furthermore, because low recombination regions often exhibit elevated interspecific differentiation [6] , [7] , [8] , disruption by potentially adaptive introgression may be particularly acute if divergent selection on variants in the region underpins differentiation. Finally, if species are very closely related and much of the interspecific divergence of their genomes is represented in low recombination regions, this detrimental effect of introgression might impact reproductive isolation directly. However, the association of differentiation with divergent selection is controversial. Low recombination regions are prone to enhanced drift, recurrent background selection and recurrent hitchhiking, which can generate similar patterns in the genome to those predicted under strong divergent selection [7] , [9] , [10] , [11] . Although usually very difficult in wild populations, recent anthropogenic selection allowed us to investigate the extent and impact of adaptive introgression into a major ‘genomic island’ region postulated to be involved in divergent selection between the Anopheles gambiae species pair [12] , [13] . The M and S forms of A. gambiae are morphologically indistinguishable and were originally identified by fixed differences in ribosomal DNA near the centromere of the X chromosome [14] . Though recently elevated to species status as A. coluzzii (M form) and A. gambiae sensu stricto (S form) [15] , for continuity with past work we retain the nomenclature of M and S, but discuss how our results bear on this formal species definition. Divergence of M and S is thought to be driven by ecological niche separation of larval habitats [16] . Differences in swarming locations have also been documented [17] , and even in mixed swarms mating is usually assortative [18] . However, M and S lack postzygotic isolation in the laboratory [19] and hybrids are found occasionally in wild populations, although this frequency varies with country [20] . Turner et al . [12] identified two large regions of the genome towards the centromeres of chromosomes X and 2L that exhibit exceptional divergence between M and S forms. This novel discovery provided evidence compatible with mosaic genome models of ecological speciation with gene flow [21] , [22] and helped to spur the field of speciation genomics. Such ‘genomic islands of divergence’ are hypothesized to arise via selection acting on a small number of physically linked variants, and grow through hitchhiking of additional physically linked adaptive and neutral loci [11] , [12] , [23] , [24] , [25] . Moreover, although hybrids may be selected against [26] , there is clear evidence for at least some contemporary gene flow extending beyond the F 1 generation throughout the range in which M and S co-occur [26] , [27] , [28] , a key assumption of mosaic genome models of ecological speciation [7] , [22] . Nevertheless, discovery of additional areas of genomic divergence [29] , [30] , [31] supported theoretical concerns [7] , [9] that the 2L and X genomic islands might be unrelated to speciation, their size arising via recurrent background selection and hitchhiking in the areas of extremely low recombination. Resolution of these competing hypotheses has been hindered by the complexity of phenotypic differences between the species pair [16] , which make laboratory studies very difficult. As a consequence, the importance of large genomic islands in the speciation process remains unclear. Malaria-transmitting mosquitoes are subjected to massive insecticidal pressure, which drives selection for rapid development of resistance [32] , [33] , [34] . Non-synonymous mutations in one of the two target sites for insecticides important in vector control, the voltage-gated sodium channel ( Vgsc ), are of particular significance. In A. gambiae the best known Vgsc mutation, L1014F , confers knockdown resistance ( kdr ) to DDT and pyrethroids via a conformational alteration which reduces binding affinity of the insecticide [35] . In West Africa, Vgsc-1014F introgressed recently from S to M forms [30] , [36] and has subsequently increased dramatically in frequency in M [33] , [37] consistent with strong anthropogenic selection [33] . The Vgsc is located within the large genomic island of divergence on chromosome arm 2L. Therefore, adaptive introgression and selection of Vgsc-1014F will result in reduced interform divergence, but the extent and impact of this genomic disruption is unknown. In A. gambiae from southern Ghana, where M and S are broadly sympatric, we show that the entire 2L genomic island introgressed with apparently negligible impact on reproductive isolation during a period of rapid Vgsc-1014F increase, suggesting that it is neither critical to speciation nor maintained by strong divergent selection. Extent and impact of kdr introgression We sequenced the whole genomes of 15 wild-caught Ghanaian A. gambiae from three groups: S homozygous for the Vgsc-1014F kdr mutation; wild-type M that lack kdr (M-wt); and M homozygous for the kdr allele that introgressed from S (M- kdr ). Comparison of M-wt and S form shows divergence across all chromosomes ( Fig. 1a ) concordant with previous low-density genome scans of Ghanaian M and S [27] , [30] and high-density single-nucleotide polymorphisms (SNPs) genotyping of samples from Mali, Burkina Faso and Cameroon [28] , [29] . However, the two large islands near the centromeres of 2L and X identified originally [12] are most prominent ( Fig. 1a ). Comparisons between the groups of samples show that over 3 Mb, representing approximately 1.5% of the genome and apparently encompassing the entire 2L island of divergence, has introgressed between species. Consequently, divergence between M- kdr and S forms in this region of the genome has been eradicated ( Fig. 1b ), and in turn high, localized differentiation between M- kdr and M-wt created by introgression ( Fig. 1c ). Beyond the 2L island the genomes of M- kdr and M-wt are minimally differentiated ( Fig. 1c ), suggesting that either only the 2L island region introgressed from F 1 hybrids, or, perhaps more likely, that larger introgressed fragments have reduced in size through back-crossing and recombination within the M form. 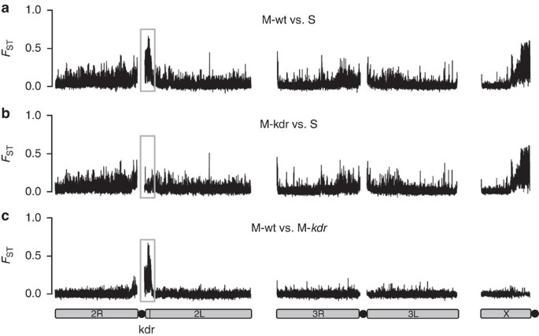Figure 1: Manhattan plots showingFST-based pairwise divergence between groupings ofA. gambiae. Plots are based on meanFSTin 100-SNP stepping windows for (a) M-wt versus S, (b) M-kdrversus S, (c) M-wt versus M-kdr.Grey boxes highlight the 2L genomic island region involved in introgression. Chromosomes are shown by solid grey bars and centromere positions by black circles. The position of thekdr(Vgsc-1014F) locus is shown on chromosome arm 2L. Figure 1: Manhattan plots showing F ST -based pairwise divergence between groupings of A. gambiae . Plots are based on mean F ST in 100-SNP stepping windows for ( a ) M-wt versus S, ( b ) M- kdr versus S, ( c ) M-wt versus M- kdr. Grey boxes highlight the 2L genomic island region involved in introgression. Chromosomes are shown by solid grey bars and centromere positions by black circles. The position of the kdr ( Vgsc-1014F ) locus is shown on chromosome arm 2L. Full size image We mapped the frequencies of M and S in larval collections from across southern Ghana ( Fig. 2 ). Overall, M and S were found at similar frequencies (55%:45%), and though relative frequencies varied considerably among locations, M and S co-occurred in 15 of the 18 collection sites. In southern Ghanaian M forms, Vgsc-1014F is now present at consistently high frequency (mean±s.d.=0.79±0.07; range=0.67–0.90), in marked contrast to when first detected in 2002 ( Fig. 3a ). This dramatic increase—to a frequency similar to that already present in S forms in 2002 (refs 38 , 39 —is indicative of strong directional selection [33] . Despite the opportunity for hybridization afforded by widespread sympatry, frequencies of M/S hybrids throughout the period of dramatic kdr increase have remained low and stable ( Fig. 3b ). This suggests (i) minimal impact of introgression of the 2L genomic island on reproductive isolation and (ii) that any divergent selection maintaining the island was much weaker than the directional selection driving the kdr mutation to high frequency. We examined whether a relatively low frequency of S forms in a collection site might limit opportunities for kdr introgression into M. However, there was no difference in current M- kdr frequencies between sites where S forms were rare (S frequency 0–0.09; kdr frequency=0.78) or those where they were common (S frequency 0.48–0.96; kdr frequency=0.82; t -test; t =0.82, P =0.41). Although relative frequencies of M and S in sampling locations may have varied during the period of kdr increase, available evidence of no current association between relative S frequencies and kdr frequency in the M form points to relatively infrequent introgression of kdr , rather than manifold introgression events. In the following sections we examine evidence that might explain how introgression of such a large, highly divergent fragment could spread so rapidly and without apparent impact on reproductive isolation via three hypotheses: (1) Only part of the 2L island introgressed, without key loci involved in reproductive isolation; (2) The 2L island is selectively unimportant as speciation is advanced and divergence is genome wide; (3) The divergence of the 2L island results from processes reducing nucleotide diversity in low recombination regions rather than contemporary divergent selection. 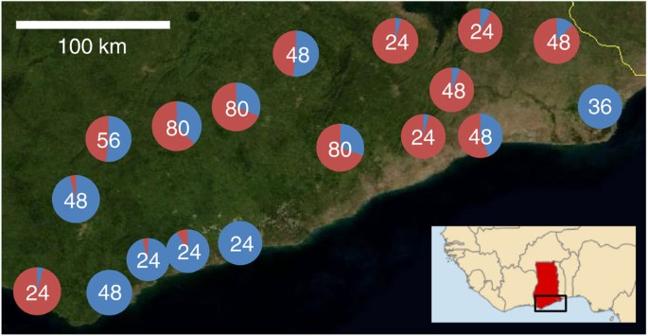Figure 2: Distribution of the M and S forms ofA. gambiaethroughout southern Ghana. Pie charts show the relative frequency of S form (shown in red) and M form (in blue), from each site (N=18) in collections made in 2011 (totalN=787). The number collected at each site is shown in the centre of each pie chart. Figure 2: Distribution of the M and S forms of A. gambiae throughout southern Ghana. Pie charts show the relative frequency of S form (shown in red) and M form (in blue), from each site ( N =18) in collections made in 2011 (total N =787). The number collected at each site is shown in the centre of each pie chart. 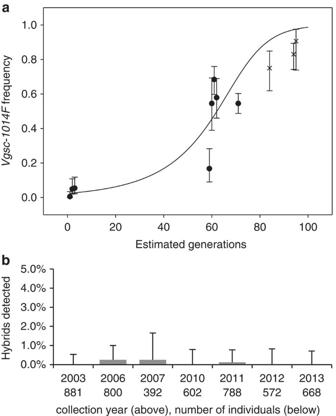Figure 3: Spread ofVgsc-1014F kdrin M forms and M/S hybridization rates. (a) Increase inVgsc-1014Ffrequency in M forms in Ghana, redrawn from the study by Lyndet al.33with permission of Oxford University Press (points shown as filled circles) with additional data points (points shown as x). (b) Hybridization rates observed over a similar collection period with error bars showing binomial 95% upper confidence intervals. Sample size for each year is shown beneath theXaxis. Full size image Figure 3: Spread of Vgsc-1014F kdr in M forms and M/S hybridization rates. ( a ) Increase in Vgsc-1014F frequency in M forms in Ghana, redrawn from the study by Lynd et al . [33] with permission of Oxford University Press (points shown as filled circles) with additional data points (points shown as x). ( b ) Hybridization rates observed over a similar collection period with error bars showing binomial 95% upper confidence intervals. Sample size for each year is shown beneath the X axis. Full size image Hypothesis 1 Visual inspection of F ST -based Manhattan plots ( Fig. 1 ) suggest that the entire 2L genomic island of divergence introgressed, but to examine this further we calculated mean pair wise nucleotide diversity (π) from the centromere across the first 5 Mb of the 2L chromosome arm (numbering on 2L starts at the centromere); a region exceeding the span of the genomic island. Neither S nor M-wt exhibited any evidence of reduced π ( Fig. 4a,b ), though the S form does experience localized lower π relative to M, possibly due to the effects of the historical sweep around Vgsc-1014F in S [33] . In contrast, and as expected in a region currently undergoing a selective sweep, the M- kdr group shows a sharp drop in π ( Fig. 4c ). However, unlike F ST ( Fig. 1b,c ), the signal from reduced nucleotide diversity does not span the entire 2L island ( Fig. 4c ). To investigate this disparity in more detail, we first identified ancestry informative loci (that is, ‘fixed’ differences between the M-wt and S samples). Loci were then classified in each individual from the M- kdr sample as homozygous M-ancestry, homozygous S-ancestry or heterozygous (mixed ancestry) in the first 5 Mb of the 2L chromosome arm ( Fig. 5 ). All M- kdr samples showed M-ancestry from approximately 3.3–5 Mb onwards, and in three of the five M- kdr individuals, S-ancestry extended unbroken from approximately 3.3 Mb back to the centromere. The other two M- kdr individuals showed near-perfect mixed ancestry in the first 1.4 Mb of the chromosome arm, with an identical transition point to homozygous S-ancestry, indicating recombination at a single breakpoint within the 2L island ( Fig. 5 ). S-ancestry did not extend across the centromere into chromosome arm 2R in any M- kdr individual ( Supplementary Fig. 1 ). The integrity of the S island in eight out of the ten M- kdr chromosomes examined and the near 50:50 mixed ancestry in the other two from the centromere to the single shared breakpoint at 1.4 Mb, suggests that recombination is recent. Thus introgression most likely did result in transfer of the entire genomic island of divergence, which extends to 3.3 Mb, with recombination only just beginning to restore the M genomic background. 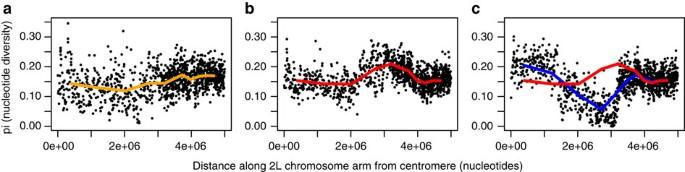Figure 4: Nucleotide diversity (π) across the first 5 Mb of chromosome arm 2L, encompassing the genomic island region. For each sample group individual points represent mean π in 100 bp stepping windows, whereas coloured lines are smoothed by using a 10 kb stepping window scale in (a) S form, (b) M-wt and (c) M-kdr, represented by the blue line, with the M-wt line (red) included for comparison. Figure 4: Nucleotide diversity (π) across the first 5 Mb of chromosome arm 2L, encompassing the genomic island region. For each sample group individual points represent mean π in 100 bp stepping windows, whereas coloured lines are smoothed by using a 10 kb stepping window scale in ( a ) S form, ( b ) M-wt and ( c ) M- kdr , represented by the blue line, with the M-wt line (red) included for comparison. 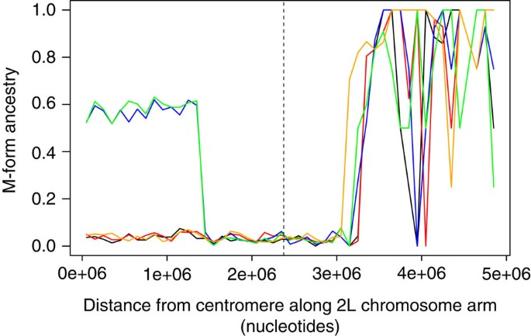Figure 5: Analysis of recombination within the introgressed 2L genomic island. Lines show proportionate M form ancestry for each individual in the M-kdrgroup based on ancestry informative markers (fully diagnostic of M and S). The black dashed line indicates the location of the voltage-gated sodium channel gene. Full size image Figure 5: Analysis of recombination within the introgressed 2L genomic island. Lines show proportionate M form ancestry for each individual in the M- kdr group based on ancestry informative markers (fully diagnostic of M and S). The black dashed line indicates the location of the voltage-gated sodium channel gene. Full size image Hypothesis 2 Lack of impact of loss of the entire 2L genomic island might be because it merely represents the tip of a continuous distribution of divergence rather than a genomic island per se . To investigate this hypothesis we first examined the genomic distribution of F ST . In spite of the appearance of widespread, indeed potentially genome wide, differentiation between M and S in the Manhattan plots ( Fig. 1a ), inter-form differentiation is generally low, with a mean autosome-wide F ST (±95%CI) of only 0.032±0.0002. Low genomic divergence, but high heterogeneity can be clearly seen from kernel density plots of the F ST distributions for each chromosome arm ( Fig. 6 ) and the associated skew and kurtosis statistics ( Supplementary Table 1 ): all M-wt versus S-chromosome arm F ST distributions are highly positively skewed and leptokurtic with long tails created by highly divergent SNPs ( Fig. 6 ). 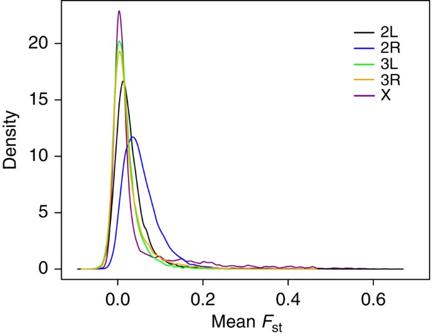Figure 6: Kernel density plots ofFSTfor M-wt versus S for each chromosome arm. Distributions of meanFST,calculated over 100-SNP stepping windows for all chromosome arms. Figure 6: Kernel density plots of F ST for M-wt versus S for each chromosome arm. Distributions of mean F ST, calculated over 100-SNP stepping windows for all chromosome arms. Full size image To facilitate precise localization of areas of marked divergence (putative genomic islands) we utilized the ancestry informative loci, this time across the whole genome (0.24% of all 13,924,420 SNPs). From the proportion of fixed differences within 50 kb windows (fixed difference, d f ) we defined non-contiguous windows significantly enriched for ancestry informative loci as distinct putative genomic islands of divergence. Plots of d f suggest the presence of genomic islands ( Fig. 7 ), albeit highly variable in size and number across chromosome arms ( Table 1 , Supplementary Data 1 ). Over 80% of the putative islands are small, comprising of three or fewer adjacent significant 50 kb windows ( Table 1 ), whereas three were very large, the 2L island (3.3 Mb) and the two adjacent pericentromeric X islands (1.45 and 4.9 Mb), which were likely merged in earlier low resolution analyses [12] , [31] . Maximum and mean d f were very strongly correlated with one another ( Supplementary Table 2 ) and with island size ( Supplementary Fig. 2a,b ), that is, islands with higher d f also tended to cover larger areas. Among islands both mean and maximum d f were significantly positively correlated with SNP frequency ( Supplementary Table S2 ), and though island size was not, it was notable that the largest islands had relatively few SNPs ( Supplementary Fig. 2c ) and also relatively few genes ( Supplementary Fig. 2d ). This contrast highlights the different patterns of polymorphism between smaller and very large islands, with the former exhibiting increasing SNP frequency with size, a relationship which breaks down for the largest islands. Our results suggest that genomic divergence between M and S is both highly heterogeneous and largely restricted to islands. Moreover, the very large islands on 2L and X remain almost as prominent as originally suggested in early low-resolution scanning [12] and contain almost 45% of all significantly differentiated windows. In summary, though islands appear both far more numerous and thus cover more of the genome than originally thought [12] , divergence appears too heterogeneous in both island size and distribution to be considered as genome wide [40] , [41] ; therefore hypothesis 2 is not supported. 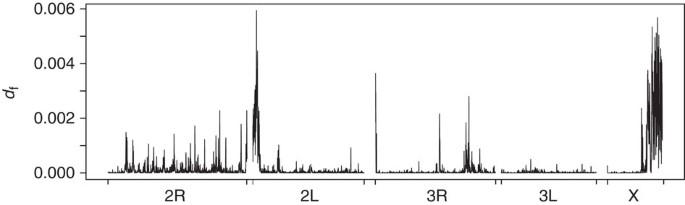Figure 7: Genomic landscape of divergence between M and S. The density of fixed differences (SNPs) between M-wt and S (df) in 50 kb stepping windows. Chromosomes and centromere position are shown by grey bars and black circles respectively; the position of thekdr Vgsc-1014Flocus is shown. Figure 7: Genomic landscape of divergence between M and S. The density of fixed differences (SNPs) between M-wt and S ( d f ) in 50 kb stepping windows. Chromosomes and centromere position are shown by grey bars and black circles respectively; the position of the kdr Vgsc-1014F locus is shown. Full size image Table 1 Size distribution of islands divergent between M and S. Full size table Hypothesis 3 Our data suggest that genomic divergence between M and S is appropriately described by an island model, albeit one involving many islands. Detailed recombination rate data are currently unavailable for the A. gambiae genome, but the location of the 2L island and the largest islands on the X chromosome near centromeres suggests that they are likely to experience reduced recombination [6] , [7] , [10] , [42] , [43] , which is consistent with their relatively low gene and SNP densities. F ST is inversely related to genetic diversity (estimated by number of segregating sites per window— Supplementary Fig. 3 ), and strong differentiation could reflect the actions of forces, other than contemporary divergent selection, that reduce diversity which is then very slow to recover in low recombination regions [7] , [11] . Consequently, we examined additional metrics for evidence of selection operating on islands, which might provide a means of partitioning historical signals of reduced diversity from recent divergent selection [7] , [9] , [11] . We first calculated Dxy [44] , a measure of absolute divergence of all nucleotide positions in a sequence, for 50 kb windows. Nevertheless, caution is required in application of Dxy, which is prone to high variance with smaller sample size, and is known to exhibit high stochastic variance among SNPs [45] , both of which might affect genome scan analyses. Consistent with, for example, the effects of background selection in low recombination regions [7] , [9] , Dxy was depressed near centromeres ( Supplementary Fig. 4 ) and peaks were not coincident with the islands identified using d f (only one out of the 436 windows which comprise the islands exceeded a 0.99th percentile of Dxy). Such observations would appear to support hypothesis 3, that the islands could reflect historical rather than contemporary selective events [7] . However, Dxy was highly positively correlated with SNP frequency of islands ( ρ =0.89, P <0.001) and also with its standard deviation within windows ( ρ =0.98, P <<0.001). Indeed, the relationship between the mean and standard deviation of Dxy is higher for islands generally, and the three very large islands (on X and 2L) show especially extreme relative standard deviation ( Fig. 8 ). In other words, the islands identified using d f did contain large values of Dxy, but many monomorphic sites (that is, a low SNP frequency) inevitably reduce values across a window, leading to exceptional variance for a given Dxy value. This will render Dxy extremely sensitive to the size of particular windows, with potential for ambiguous interpretation. Therefore, if covariates affecting Dxy are considered it could not usefully provide discrimination of competing hypotheses for our dataset. Moreover, we note a high correlation ( r =–0.5) between sequence depth and Dxy, suggesting sensitivity to sequencing error. 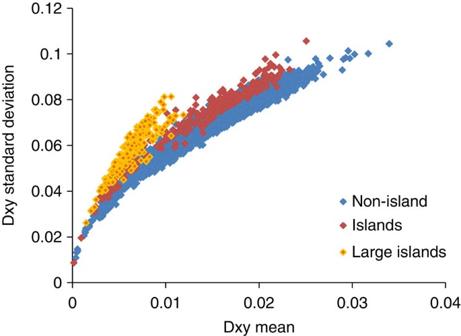Figure 8: Scatterplot of absolute divergence, Dxy, plotted against its standard deviation. Points are means for every 50 kb window in the genome, with colours denoting windows from genomic islands of divergence (red), those from the three largest islands of divergence (those over 1 Mb in size), two on the X chromosome and one on 2L (yellow) and the windows from the rest of the genome (blue). Figure 8: Scatterplot of absolute divergence, Dxy, plotted against its standard deviation. Points are means for every 50 kb window in the genome, with colours denoting windows from genomic islands of divergence (red), those from the three largest islands of divergence (those over 1 Mb in size), two on the X chromosome and one on 2L (yellow) and the windows from the rest of the genome (blue). Full size image Second we calculated Tajima’s D [46] , again for 50 kb windows; extreme values of D result from an imbalance between pairwise nucleotide diversity and the number of segregating sites, with negative values potentially indicating directional selection and high values, balancing selection. In contrast to Dxy, a low correlation between sequence depth and Tajima’s D was found ( r =0.19). There was no signal of directional selection around the 2L island in any group ( Fig. 9 ), with S forms actually exhibiting the highest positive values of Tajima’s D within the 2L island, indicative of balancing selection ( Supplementary Fig. 5 ). This counterintuitive result seems unlikely to reflect balancing selection, but is concordant with theoretical expectations for a positive Tajima’s D signal [47] arising from a secondary selective sweep of the region, which overlays an earlier sweep likely driven by Vgsc-1014F . The recently discovered resistance allele Vgsc-1575Y [34] could provide a plausible candidate, as all the S-form individuals sequenced were N1575Y heterozygotes, although at around 3 Mb on 2L, the peak of Tajima’s D is offset from the Vgsc . 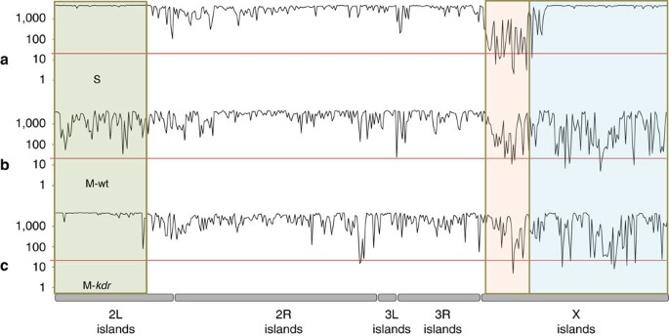Figure 9: Evidence of directional selection from Tajima’s D across all genomic islands in each group. Plots show ranks of Tajima’s D negative values (lower=more negative) for the 438 significant windows comprising islands, arrayed in order of physical position on each chromosome arm for the three sample groups: (a) S form, (b) M-wt and (c) M-kdr. Ranks are initially calculated across all 4,612 windows within each group, but only island window are shown. The red line shows the two-tailed lower 99th percentile rank used as a threshold for extreme values. Windows within the major 2L island and in the pair of very large islands of divergence on the X chromosome are highlighted in shaded boxes. Figure 9: Evidence of directional selection from Tajima’s D across all genomic islands in each group. Plots show ranks of Tajima’s D negative values (lower=more negative) for the 438 significant windows comprising islands, arrayed in order of physical position on each chromosome arm for the three sample groups: ( a ) S form, ( b ) M-wt and ( c ) M- kdr . Ranks are initially calculated across all 4,612 windows within each group, but only island window are shown. The red line shows the two-tailed lower 99th percentile rank used as a threshold for extreme values. Windows within the major 2L island and in the pair of very large islands of divergence on the X chromosome are highlighted in shaded boxes. Full size image Highly negative values of Tajima’s D were almost entirely absent from the autosomes of M and S; though peaks were found throughout both of the two centromere-proximal X chromosome islands in M forms ( Fig. 9 ). In S, there was a notable clustering of negative Tajima’s D peaks centred around 18.5 Mb, with extreme values (exceeding a two-tailed 99% threshold) just extending into the beginning of the largest X island ( Fig. 9 ) and thus clearly offset from peak interform divergence on X ( Figs 1 and 7 ). Coincident outlying negative values were also found in the smaller island region within both M groups. Gene annotation term enrichment analysis identified a significant overrepresentation of genes linked with chitin synthesis genes in this region ( Supplementary Table 3 ). The negative Tajima’s D signals throughout the largest X islands in both M groups, but not in S, suggest selection potentially acting within M forms rather than divergent selection acting on both M and S, as found in the smaller X island. The relationship between Dxy and its variance suggests unreliability because of extreme dependence on window size and a concerning potential for sensitivity to sequencing error. Tajima’s D suggested some concordance of divergent regions with selection, though the likely conflation of signals within the 2L island region highlights that problems can occur with interpretation. However, Tajima’s D yielded some signals of selection for each of the large X islands. In particular, the secondary island region on X, which lies outside of the pericentromeric heterochromatin region of extreme low recombination [43] , is both significantly divergent between M and S, and shows evidence of contemporary directional selection operating within M and S, supporting a novel hypothesis of involvement in ongoing divergence. In summary, though hypothesis 3 is difficult to disprove conclusively, Tajima’s D provided evidence of ongoing selection on the X islands (if not for the 2L island), and highlights the utility of combining multiple metrics in candidate region discovery. In this study we investigated a case of introgression between the most recently diverged species within the A. gambiae complex. The adaptive nature of the Vgsc1014F mutation is clearly evident from its significant association with insecticide resistance [34] and its dramatic rate of increase in A. gambiae M forms. Introgression of Vgsc1014F from S to M forms has also been documented in Benin [36] , Cameroon [48] and Burkina Faso [37] , with a similarly rapid increase in frequency observed in the latter. Moreover, though not explicitly considered by the authors, temporal variation in numbers of hybrids and back-crosses detected in a longitudinal study of a single village in Mali [26] might be linked to selection for introgression of Vgsc-1014F into M forms, rather than relaxed selection against hybrids and back-crosses linked to other unknown environmental variations [26] . The present data are unique in demonstrating the genomic extent of introgression. However, studies of introgression from Mali and Cameroon, albeit based on only one or two SNPs in the 2L genomic island region outside of the Vgsc [26] , [27] , and also the variety of locations from which kdr introgression has been recorded, suggest that our results are very unlikely to be restricted to southern Ghana. Given the location of the Vgsc gene in the 2L pericentromeric region, which is thought to exhibit low recombination [29] , [49] , we hypothesized that a relatively extensive area might be affected by the selective sweep. In fact, the impacted area proved to be huge, exceeding 3 Mb (1.5% of the genome), and spanned the entirety of one of the two most prominent genomic islands of divergence between M and S. Coupled with hybridization data collected during the period of Vgsc1014F increase in M forms, this provided a natural test of whether the loss of a major genomic island of divergence reduces the reproductive isolation of M and S, as might be expected if the island contained genes critical to the speciation process; that is, a ‘speciation island’ [12] . Our results do not support the designation of the 2L genomic island of divergence as a speciation island. M and S forms are extensively sympatric across southern Ghana, presenting widespread opportunity for hybridization. Yet hybridization rates appear stable throughout the period of rapid increase of introgressed Vgsc1014F to high frequency in M form populations across southern Ghana. It would appear that transfer of the entire island has had no discernible impact on reproductive isolation, allowing effective co-option of the adaptive Vgsc-1014F mutation into the M genomic background via adaptive introgression. The large pericentromeric speciation islands on separate chromosomes (X, 2L and 3L) are usually in strong linkage disequilibrium, which could imply epistatic selection [10] , [31] . If this were the case, it seems unlikely that the genome of M forms could tolerate such massive disruption without a major loss of fitness. By contrast, our results suggest that any M form fitness cost is overcome by the increase in fitness from gaining the Vgsc-1014F mutation. It would seem therefore, that any selective importance of the 2L island of divergence does not arise from its impact on reproductive isolation, and that it is not currently involved in speciation. Though some past involvement in divergence cannot be ruled out, our results highlight that large areas of interform divergence, however eye-catching, are not necessarily under selective forces proportional to their size. Reduced haplotypic diversity in the Vgsc of S forms is evidence for recent selection [33] , which, before introgression of the Vgsc-1014F mutation and increase to high frequency in M forms, would have resulted in increased divergence. Although interpretation of the strong Tajima’s D signal of selection on 2L was ambiguous, and given low recombination in the 2L island, it is possible that a portion extending some way beyond the Vgsc might have been subjected to the sweep of Vgsc-1014F . This poses the question of whether M and S divergence on 2L is simply a result of selection operating within S forms. Selection on Vgsc-1014F can be discounted as a general explanation because divergence in this region was first documented from comparison of M and S, which both lacked the Vgsc-1014F mutations [12] . Selection within S alone is also not supported by comparative patterns of nucleotide diversity in the island region, levels of which are broadly similar in M-wt and S across the island region despite the historical selective sweeps in S [33] , [34] ( Fig. 4a,b ). Apart from recent selection on Vgsc-1014F , is the 2L island under any contemporary directional selection at all or is its size an artefact of background selection? Unfortunately, the additional metrics we applied (Dxy and Tajima’s D) did not allow separation of these hypotheses but selection on Vgsc-1014F provides some additional insight. Given the very rapid increase in Vgsc-1014F frequency in M forms following introgression, any negative fitness consequences resulting from loss of alleles under selection within the 2L island must have been outweighed by insecticidal selection on Vgsc-1014F , for which we have estimated a selection coefficient of s =0.16 (ref. 33 ). From the size of the introgressed fragment, it is now apparent that this represents a net estimate for the 3.3 Mb 2L island of divergence, rather than Vgsc-1014F alone. Thus, either selection on Vgsc-1014F is much stronger than initially estimated or the total selection acting on all variants within the 2L island of divergence is weak. If selection on such a large island appears weak, it is natural to question the importance of the other, often small, islands throughout the genome and whether reduced recombination plays a key role in their formation [8] . SNP frequency data do not support the latter for many of the smaller islands, which, in contrast to the very large islands, often showed quite high densities of segregating sites, at odds with the expectation for a low recombination region. Nevertheless, differentiation of so many islands seems puzzling unless they are by-products of genome-wide divergence, which does not appear to fit their heterogeneity in size and distribution. To account for the genomically widespread differences between M and S, when there is clear evidence for recent gene flow, Reidenbach et al . [28] proposed an ‘extrinsic’ environmental hypothesis. In this scenario, hybridization occurs in infrequent bursts during unusual environmental conditions, with strong selection against introgressed individuals when typical conditions return [28] . Recent data from a time series study in a Malian village appear consistent with this hypothesis [26] , though as noted above Vgsc-1014F introgression might also be involved. An alternative, and not mutually exclusive ‘intrinsic’ hypothesis, is that the nature of the genomic landscape of divergence provides permissiveness to gene flow. Selection dispersed across many islands is likely to be weak for the majority of loci, potentially enabling resilience to temporary loss of (weakly selected) islands until they can be restored by back-crossing. Searching for ‘individual speciation genes’ in such a landscape will thus be difficult because of low selection coefficients and frequent lack of correspondence between significant divergence and functionality. Our results provide a natural ‘loss of function’ test of the 2L island, which bears many similarities in terms of likely recombination profile, polymorphism and divergence to the only other exceptionally large islands, located on the X chromosome. We think it is unwise to extrapolate from these commonalities a similar lack of importance for the X islands in speciation between M and S. X (or Z) chromosomes evolve relatively quickly owing to reduced effective population size and are known to be critically involved in the development of reproductive isolating mechanisms between many species [50] , including other, less closely related members of the A. gambiae species complex [51] , [52] . Moreover, and although proof of a speciation island must come from demonstrable function, Tajima’s D, F ST and d f all provide signals consistent with selection acting around 17–19 Mb on the X chromosome in both M and S, and perhaps further towards the centromere in M forms. The signal of selection found in both M and S was primarily focused on the smaller of the two major X islands, the physical distance of which from the centromere may make it more likely that selection rather than just low recombination preserves its large size. Interestingly, while the largest island on X is always present when comparing M and S, this secondary X island area is absent from locales such as Guinea-Bissau, The Gambia and Senegal exhibiting exceptionally high hybridization rates [27] , [53] . Follow-up studies on the role of this genomic region are warranted. A multi-locus, resilient genomic architecture of divergence presents an interesting paradox for speciation theory. Typically, the presence of substantial gene flow has been viewed as a signal of early-stage incipient speciation [22] , some way from the degree of reproductive isolation at which organisms might be recognized as ‘good species’. However, it is becoming recognized now that gene flow between closely related ‘good species’ is extremely widespread [40] , [54] . If selection is spread across numerous loci this may effectively provide intrinsic redundancy, and interspecific gene flow may actually be a long-lasting, stable state. A genomic landscape of generally weak but highly heterogeneous differentiation, though perhaps far from a highly differentiated ‘end point’ [40] expected for species, may be an important stage in genomic divergence, which can allow both adaptive introgression and protection of reproductive isolation. The molecular forms have recently been reclassified as A. gambiae s.s. and Anopheles coluzzii [15] , based primarily on evidence of reproductive isolation from relatively widespread genomic differentiation [28] , [29] , [55] and partial ecological niche partitioning [56] , [57] . While we do not interpret our data as revealing truly genome-wide divergence, under either the ‘extrinsic’ or ‘intrinsic’ hypotheses outlined above, our results support this reclassification of M and S forms as species. Collections Adult female mosquitoes used subsequently for whole-genome sequencing were collected by aspiration from southern Ghana during the summer of 2007. Six locations ( Supplementary Table 4 ) were sampled to yield five A. gambiae S form (individuals homozygous for the Vgsc-1014F mutation) and ten A. gambiae M form (five individuals homozygous for the wild-type 1014 L and five homozygous for the introgressed Vgsc-1014F mutation). 1014F is close to fixation in A. gambiae S form populations in this region, so no homozygote 1014 L individuals were available. Multiple collection locations were necessary due to a sequencing protocol that required a high yield of extracted DNA. Before extraction all samples were stored dry over silica. Data for M/S hybrid frequencies in southern Ghana were collated from collections we have described elsewhere [30] , [38] , [39] , [58] , [59] . DNA extraction and sequencing After morphological identification as A. gambiae s.l. , DNA was extracted from dried whole bodies using the DNeasy extraction kit (Qiagen). Species (within A. gambiae s.l. ) were identified using a standard PCR diagnostic assay [60] , with subsequent identification of molecular forms using the SINE diagnostic method [61] . As Ghanaian sampling was concerned with kdr introgression, these 15 individuals were also genotyped for the presence of the voltage-gated sodium channel mutation Vgsc-1014F using a TaqMan assay [62] . DNA quantification was carried out using Quant-iT PicoGreen dsDNA fluorimetric assays (Invitrogen), taking the mean concentration from two technical replicates. Sample libraries were cloned with 200–300 bp inserts, and 76 bp paired-end sequencing was conducted using an Illumina High Seq 2000 by the Wellcome Trust Sanger Institute. Reads were aligned to the AgamP3 reference genome [63] using BWA [64] ; 82–90% of read pairs per sample successfully aligned to the reference sequence, giving a median read depth per sample of 7–20x. Variant calling was conducted using SAMtools mpileup and BCFtools to produce a raw vcf file, which was filtered using vcfutils.pl varFilter-D100 (ref. 65 ). Non-biallelic SNP loci were removed using VCFtools [66] . Sequenced individuals were re-checked for read depth, particularly in regions of interest, and molecular form was validated in the genome sequence data via presence/absence of the SINE insertion [61] using LookSeq [67] . Statistical analyses Genomic divergence between mosquito sample groups and pairwise nucleotide diversity within groups were calculated for every SNP using VCFtools version 0.1.9.0 (ref. 66 ) (commands) via the Weir and Cockerham estimator of F ST (- -weir-pop-fst) and π (- -site-pi), respectively. ‘Fixed’ differences in F ST between the S and M-wild-type sample groups were identified and used (1) as ancestry informative markers to study localized recombination in the M- kdr group, and (2) to estimate the proportion of d f (ref. 68 ) within non-overlapping 50 kb windows. This represents an arbitrary size that simply represents a balance between resolution and minimizing impacts of any SNP calling errors, and is not tailored to any specific detailed recombination map as this is unavailable for A. gambiae . Plots of F ST , d f and π against chromosomal position were produced from means of windows with the statistical software package R [69] and custom Perl and R scripts. A 100-SNP stepping window size was chosen to visualize F ST because this has been shown to produce accurate estimates of Weir and Cockerham’s F ST from low sample sizes [70] . To identify putative genomic islands of divergence, we tested for exceptional values of d f by simulating 100,000 Poisson distributions based on the actual number of windows and ancestry informative markers and applying a window-specific threshold scaled according to the SNP frequency within the window. As a conservative threshold for identification of clustering within a window we applied a Bonferroni-corrected upper percentile limit for d f from simulations: only observed d f values exceeding this were considered significant. Adjacent significant windows were considered part of the same island; however, we considered islands as continuous if a nonsignificant window intervened between significant windows, but this exceeded the upper 0.8 percentile limit of simulated d f . Kernel plots and associated skewness and kurtosis statistics were used to study the density distributions of F ST values for each SNP on each chromosome and were calculated and plotted using custom Perl scripts and R (ref. 69 ). Additional metrics to study variation in the pairwise polymorphic site-frequency spectrum between individuals within a sample and absolute divergence between samples were calculated as Tajima’s D [46] and Dxy [45] , respectively, using custom Perl scripts and R (ref. 69 ). Sequence data was ‘haploidized’ for estimation of these parameters (following Ellegren et al . [68] ) by randomly assigning alleles at heterozygous positions. Spearman correlation coefficients between descriptive statistics (none of which were normally distributed) for islands were calculated using SPSS v20 (IBM, Armonk, NY). How to cite this article: Clarkson, C.S. et al . Adaptive introgression between Anopheles sibling species eliminates a major genomic island but not reproductive isolation. Nat. Commun. 5:4248 doi: 10.1038/ncomms5248 (2014). Accession codes: The 15 A. gambiae whole-genome sequences have been deposited in the European Nucleotide Archive database under the accession codes ERS012670 to ERS012684 .